Correspondence:SEMA4Avariation and risk of colorectal cancer 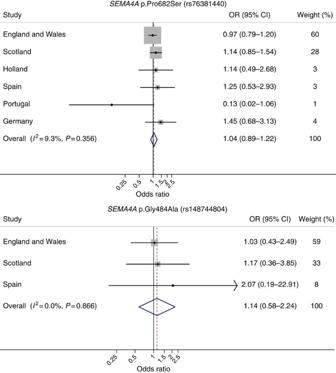Figure 1: Forest plot of association between rs148744804 and rs76381440SEMA4Agenotypes and colorectal cancer risk. Studies were weighted according to the inverse of the variance of the log of the OR calculated by unconditional logistic regression. Meta-analysis under a fixed-effects model was conducted using standard methods. Cochran’sQstatistic to test for heterogeneity and theI2statistic to quantify the proportion of the total variation due to heterogeneity were calculated. Horizontal lines indicate 95% confidence intervals (CIs). Boxes indicate odds ratio (OR) point estimate; its area is proportional to the weight of the study. Diamond (and broken line) indicates overall summary estimate, with CI given by its width. Unbroken vertical line indicates null value (OR=1.0). How to cite this article : Kinnersley, B. et al . Correspondence: SEMA4A variation and risk of colorectal cancer. Nat. Commun . 7:10611 doi: 10.1038/ncomms10611 (2016).